Genome-wide association and transcriptome studies identify target genes and risk loci for breast cancer Genome-wide association studies (GWAS) have identified more than 170 breast cancer susceptibility loci. Here we hypothesize that some risk-associated variants might act in non-breast tissues, specifically adipose tissue and immune cells from blood and spleen. Using expression quantitative trait loci (eQTL) reported in these tissues, we identify 26 previously unreported, likely target genes of overall breast cancer risk variants, and 17 for estrogen receptor (ER)-negative breast cancer, several with a known immune function. We determine the directional effect of gene expression on disease risk measured based on single and multiple eQTL. In addition, using a gene-based test of association that considers eQTL from multiple tissues, we identify seven (and four) regions with variants associated with overall (and ER-negative) breast cancer risk, which were not reported in previous GWAS. Further investigation of the function of the implicated genes in breast and immune cells may provide insights into the etiology of breast cancer. Breast cancer is the most commonly diagnosed malignancy and most frequent cause of cancer-related mortality in women [1] . Genome-wide association studies (GWAS) have detected more than 170 genomic loci harboring common variants associated with breast cancer risk, including 20 primarily associated with risk of ER-negative disease [2] , [3] . Together, these common variants account for 18% of the two-fold familial relative risk of breast cancer [2] . To translate GWAS findings into an improved understanding of the biology underlying disease risk, it is essential to first identify the target genes of risk-associated variants. This is not straightforward because most risk variants lie in non-coding regions, particularly enhancers, many of which do not target the nearest gene [4] . To help with this task, we recently developed a pipeline that identifies likely target genes of breast cancer risk variants based on breast tissue-specific genomic data, such as promoter–enhancer chromatin interactions and expression quantitative trait loci (eQTL) [2] . Using this approach, called INQUISIT, we identified 689 genes as potential targets of the breast cancer risk variants. However, it is likely that at least some breast cancer risk variants modulate gene expression in tissues other than breast, which were not considered by INQUISIT; for example, breast cancer risk variants are enriched in histone marks measured in adipose tissue [2] . On the other hand, the immune system also plays a role in the elimination of cancer cells [5] so it is possible that some breast cancer risk variants influence the expression of genes that function in the immune system. The first aim of this study was to identify additional likely target genes of the breast cancer risk variants identified by the Breast Cancer Association Consortium [2] , [3] using information on eQTL in multiple relevant tissue types: adipose, breast, immune cells, spleen, and whole-blood. The second aim was to identify previously unreported risk loci for breast cancer by formally integrating eQTL information across tissues with results from the GWAS [2] , [3] using EUGENE, a recently described gene-based test of association [6] , [7] , that is conceptually similar to other transcriptome-wide association study (TWAS) approaches, such as PrediXcan [8] . Gene-based analyses would be expected to identify previously unreported risk loci if, for example, multiple independent eQTL for a given gene are individually associated with disease risk, but not at the genome-wide significance level used for single-variant analyses. Predicted target genes of overall breast cancer risk variants Using approximate joint association analysis implemented in GCTA [9] (see Methods), we first identified 212 variants that were independently associated (i.e. with GCTA-COJO joint analysis P < 5 × 10 −8 ) with breast cancer in a GWAS dataset of 122,977 cases and 105,974 controls [2] (Supplementary Data 1 ). Of note, 20 of these variants reached genome-wide significance in the joint, but not in the original single-variant, association analysis; that is, they represent secondary signals that were masked by the association with other nearby risk variants, as described previously [9] . We extracted association summary statistics from 117 published eQTL datasets identified in five broad tissue types: adipose, breast, individual immune cell types, spleen and whole-blood (Supplementary Data 2 ). For each gene and for a given eQTL dataset, we identified cis eQTL (within 1 Mb of gene boundaries) in low linkage disequilibrium (LD; r 2 < 0.05) with each other, and with an association with gene expression significant at a conservative significance threshold of 8.9 × 10 −10 . We refer to these as “sentinel eQTL”. The mean number of sentinel eQTL per gene ranged from 1.0 to 2.9 across the 117 eQTL datasets considered, which varied considerably in sample size and number of genes tested (Supplementary Data 2 ). When we intersected the list of variants from the joint association analysis and the list of sentinel eQTL from published datasets, we identified 46 sentinel risk variants that were in high LD ( r 2 > 0.8) with one or more sentinel eQTL, implicating 88 individual genes at 46 loci as likely targets of breast cancer risk variants (Supplementary Data 3 and 4 ). Twenty-five risk variants had a single predicted target gene, 10 had two, and 11 had three or more (Supplementary Data 5 ). Of the 88 genes, 75 (85%) were identified based on eQTL from whole-blood, 10 (11%) from immune cells ( PEX14 , RNF115 , TNNT3 , EFEMP2 , SDHA , AP4B1 , BCL2L15 , BTN3A2 , HIST1H2BL , SYNE1 ), and three (4%) exclusively from adipose tissue ( ZNF703 , HAPLN4 , TM6SF2 ) (Supplementary Data 4 ). Only four sentinel risk variants were in LD with a sentinel eQTL in breast tissue (for ATG10 , PIDD1 , RCCD1 , and APOBEC3B ); all were also eQTL in whole-blood and immune cells. However, it is noteworthy that an additional 29 sentinel eQTL listed in Supplementary Data 3 had a modest, yet significant association with the expression of the respective target gene in breast tissue (GTEx V7, n = 251), suggesting that larger eQTL datasets of this tissue will be informative to identify the target genes of sentinel risk variants. A total of 62 genes were included in the list of 925 targets predicted in the original GWAS using INQUISIT [2] , while 26 genes represent previously unreported predictions (Supplementary Data 5 ). Regional association plots for these 26 genes are presented in Supplementary Fig. 1 , with three examples shown in Fig. 1 . Fig. 1 Examples of previously unreported target gene predictions at known breast cancer risk loci. Variants are represented by points colored according to the LD with the sentinel risk variant (red: ≥0.8, orange: 0.6–0.8, green: 0.4–0.6, light blue: 0.2–0.4, and dark blue: <0.2). Sentinel risk variants (triangles) were identified based on joint association analysis [9] . Figure shows on the y -axis the evidence for breast cancer association (−log 10 of the P -value in the original published GWAS results [2] , obtained in that study using an inverse-variance meta-analysis), and on the x -axis chromosomal position. Gene structures from GENCODE v19 gene annotations are shown and the predicted target genes shown in red. a The sentinel risk variant at this locus (rs875311) was in LD with sentinel eQTL for CFL1 (in whole blood) and for EFEMP2 (in CD8 + T cells only). b The sentinel risk variant (rs11049425, target gene: CCDC91 ) represents a secondary association signal in this region. c The sentinel risk variant at this locus (rs8105994) is in LD with sentinel eQTL for two previously unreported target gene predictions ( AC010335 . 1 and LRRC25 ) and four previously predicted targets ( CTD-3137H5 . 1 , ELL , PGPEP1 and SSBP4 ; (Supplementary Data 5). 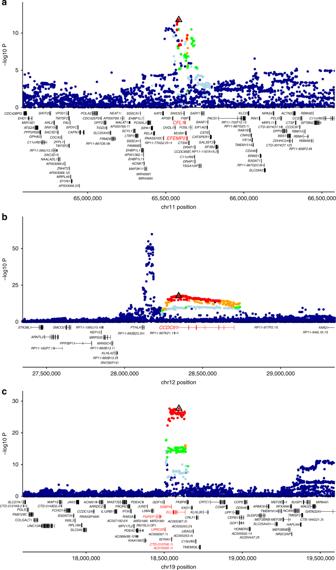Fig. 1 Examples of previously unreported target gene predictions at known breast cancer risk loci. Variants are represented by points colored according to the LD with the sentinel risk variant (red: ≥0.8, orange: 0.6–0.8, green: 0.4–0.6, light blue: 0.2–0.4, and dark blue: <0.2). Sentinel risk variants (triangles) were identified based on joint association analysis9. Figure shows on they-axis the evidence for breast cancer association (−log10of theP-value in the original published GWAS results2, obtained in that study using an inverse-variance meta-analysis), and on thex-axis chromosomal position. Gene structures from GENCODE v19 gene annotations are shown and the predicted target genes shown in red.aThe sentinel risk variant at this locus (rs875311) was in LD with sentinel eQTL forCFL1(in whole blood) and forEFEMP2(in CD8+T cells only).bThe sentinel risk variant (rs11049425, target gene:CCDC91) represents a secondary association signal in this region.cThe sentinel risk variant at this locus (rs8105994) is in LD with sentinel eQTL for two previously unreported target gene predictions (AC010335.1andLRRC25) and four previously predicted targets (CTD-3137H5.1,ELL,PGPEP1andSSBP4; (Supplementary Data 5). Regional association plots for the remaining target gene predictions for overall breast cancer (Supplementary Data3) are provided in Supplementary Figure1 Regional association plots for the remaining target gene predictions for overall breast cancer (Supplementary Data 3 ) are provided in Supplementary Figure 1 Full size image Directional effect of gene expression on breast cancer risk For the 88 genes identified as likely targets of breast cancer risk variants, we studied the directional effect of genetically-determined gene expression on disease risk, based on the sentinel eQTL that was in LD with the sentinel risk variant. For each gene, we first determined whether the eQTL allele that was associated with reduced breast cancer risk was associated with higher or lower target gene expression. Of the 77 genes for which this information could be obtained (detailed in Supplementary Data 4 ), the protective allele was associated with lower expression for 43 genes (e.g. GATAD2A , FAM175A , KCNN4 , and CTB-161K23 . 1 ) and higher expression for 28 genes (e.g. RCCD1 , ATG10 , ELL , and TLR1 ) (summarized in Table 1 and Supplementary Data 6 ). For the remaining six genes ( ADCY3 , AMFR, APOBEC3B, CCDC127, HSPA4 , and MRPS18C ), conflicting directional effects were observed across different tissues, and so the interpretation of results is not straightforward. Table 1 Directional effect of genetically determined gene expression on disease risk for predicted target genes of breast cancer sentinel risk variants Full size table Directional effect based on information from multiple eQTL In the previous analysis, the directional effect of gene expression on disease risk was assessed based on a single eQTL at a time.However, the expression of most genes is associated with multiple independent eQTL, which may not have the same directional effect on disease risk. To address this limitation, we assessed if results from the single QTL analyses above were recapitulated by considering information from multiple eQTL using S-PrediXcan [10] . We applied this approach to the same GWAS results [2] and used transcriptome prediction models from whole-blood, generated based on data from the Depression Genes and Network study ( n = 922 [11] ) and GTEx ( n = 369). We used SNP prediction models for gene expression in whole-blood because most genes (75 of 88) were identified as likely targets based on eQTL information from this tissue. Results from this analysis are presented in Supplementary Data 7 . The predicted directional effect of gene expression on disease risk was available in both the single eQTL and S-PrediXcan analyses for 48 of the 88 likely target genes. For 42 of those 48 genes (88%) the two predictions matched, supporting a consistent directional effect across multiple eQTL of the same gene. The inconsistent results observed for the remaining six genes were likely caused by technical biases (possible explanations in Supplementary Data 7 ). Similar findings were obtained when considering whole-blood transcriptome prediction models based on data from the GTEx consortium (Supplementary Data 7 ). Overall, these results indicate very good agreement between the directional effect of gene expression on disease risk obtained using information from individual or multiple eQTL. Target gene predictions supported by functional data The 88 genes identified represent target predictions that should be experimentally validated, as outlined previously [12] . To help prioritize genes for functional follow-up, we identified a subset for which publicly available functional data supported the presence of either (i) chromatin interactions between an enhancer and the gene promoter [4] , [13] , [14] , [15] ; or (ii) an association between variation in enhancer epigenetic marks and variation in gene expression levels [16] , [17] , [18] , [19] . We only considered enhancers that overlapped a sentinel risk variant (or a proxy with r 2 > 0.80) and restricted our analysis to blood cells (Supplementary Data 8 ), given that most target genes were identified based on eQTL data from whole-blood. We found that 25 (28%) of the 88 target gene predictions were supported by functional data (Supplementary Data 9 ). Previously unreported risk loci for breast cancer The second major goal of this study was to identify previously unreported risk loci for breast cancer using gene-based association analyses. We first used approximate conditional analysis implemented in GCTA [9] to adjust the GWAS results [2] (Fig. 2a ) for the effects of the 212 variants that had a significant independent association with overall breast cancer. As expected, in the resulting adjusted GWAS no single variant had a genome-wide significant association (i.e. all had a GCTA-COJO conditional association P > 5 × 10 −8 ; Fig. 2b ). We then applied the EUGENE gene-based approach [6] , [7] to the adjusted GWAS results, considering in a single association analysis cis eQTL identified in five broad tissue types: adipose, breast, immune cells, spleen, and whole-blood (Supplementary Data 10 ). That is, we did not perform a separate gene-based analysis for each tissue, but rather a single analysis that considers all eQTL reported across the five tissues. Fig. 2 Manhattan plots summarizing association results for overall breast cancer. a Association results (−log 10 of the P -value obtained using an inverse-variance meta- analysis) from the single-variant GWAS originally reported by Michailidou et al. [2] . b Single-variant GWAS adjusted for 212 sentinel risk variants and LD-score intercept; P -values were obtained with the GCTA-COJO joint analysis. 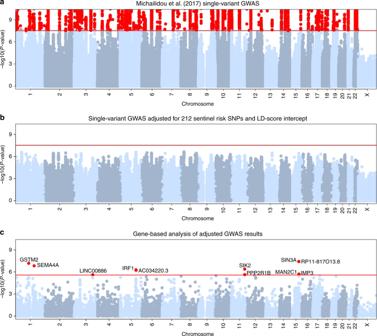Fig. 2 Manhattan plots summarizing association results for overall breast cancer.aAssociation results (−log10of theP-value obtained using an inverse-variance meta- analysis) from the single-variant GWAS originally reported by Michailidou et al.2.bSingle-variant GWAS adjusted for 212 sentinel risk variants and LD-score intercept;P-values were obtained with the GCTA-COJO joint analysis.cGene-based analysis of adjusted GWAS results;P-values were obtained with the EUGENE gene-based test of association c Gene-based analysis of adjusted GWAS results; P -values were obtained with the EUGENE gene-based test of association Full size image Of the 19,478 genes tested (full results provided as Supplementary Material), 11 had a significant gene-based association after correcting for multiple testing (EUGENE P < 0.05/19,478 = 2.5 × 10 −6 ; Table 2 ; Fig. 2c ). The specific eQTL included in the gene-based test for each of these 11 genes, which were located in six loci >1 Mb apart, are listed in Supplementary Data 10 . Regional association plots for the 11 genes are presented in Supplementary Fig. 2 , with three examples shown in Fig. 3 . Except for the MAN2C1 locus [20] , these loci have not previously been identified by GWAS and thus represent putative breast cancer susceptibility loci. Table 2 Risk loci for breast cancer identified in the EUGENE gene-based analysis but not in previous GWAS Full size table Fig. 3 Examples of significant gene-based associations at loci not previously reported in breast cancer GWAS. Variants are represented by points colored according to the LD with the sentinel risk variant (red: ≥0.8, orange: 0.6–0.8, green: 0.4–0.6, light blue: 0.2–0.4, and dark blue: <0.2). Sentinel eQTL included in the EUGENE analysis (triangles) were identified from published eQTL studies of five different tissue types. Figure shows on the y -axis the evidence for breast cancer association (−log 10 of the P -value in the published GWAS after adjusting for the association with the sentinel risk variants using the COJO-COND test, and the LD-score intercept), and on the x -axis chromosomal position. The sentinel eQTL most associated with breast cancer risk is depicted by a black triangle; other sentinel eQTL included in the gene-based test are depicted by red triangles. Gene structures from GENCODE v19 gene annotations are shown and the predicted target genes shown in red. a – c show examples of three previously unreported loci which respectively implicate PPP2R1B , IMP3 and GSTM2 as candidate breast cancer susceptibility genes. Regional association plots for the remaining eight gene- based associations are provided in Supplementary Figure 2 Full size image For most (9 of 11) genes identified, the association P -value obtained with the gene- based test was more significant than the P -value obtained with the individual eQTL most associated with disease risk, indicating that multiple sentinel eQTL for the same gene were associated with disease risk (range 2–6 associated eQTL per gene; Table 2 ). For example, the EUGENE gene-based P -value for GSTM2 was 6.6 × 10 −8 , while the best individual eQTL showed more moderate association with breast cancer risk (GCTA-COJO conditional association P = 4.1 × 10 −5 ; five of the 14 sentinel eQTL tested for this gene were nominally associated with disease risk (Supplementary Data 11 ). We also studied the predicted directional effect of gene expression on disease risk, as described above for target genes of known breast cancer risk variants. 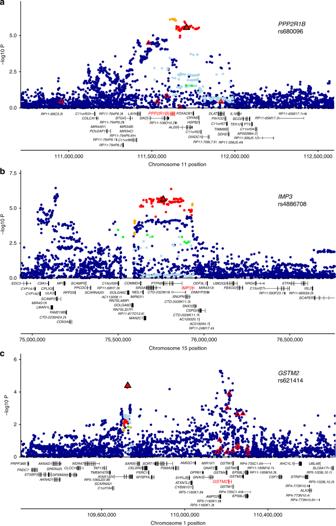Fig. 3 Examples of significant gene-based associations at loci not previously reported in breast cancer GWAS. Variants are represented by points colored according to the LD with the sentinel risk variant (red: ≥0.8, orange: 0.6–0.8, green: 0.4–0.6, light blue: 0.2–0.4, and dark blue: <0.2). Sentinel eQTL included in the EUGENE analysis (triangles) were identified from published eQTL studies of five different tissue types. Figure shows on they-axis the evidence for breast cancer association (−log10of theP-value in the published GWAS after adjusting for the association with the sentinel risk variants using the COJO-COND test, and the LD-score intercept), and on thex-axis chromosomal position. The sentinel eQTL most associated with breast cancer risk is depicted by a black triangle; other sentinel eQTL included in the gene-based test are depicted by red triangles. Gene structures from GENCODE v19 gene annotations are shown and the predicted target genes shown in red.a–cshow examples of three previously unreported loci which respectively implicatePPP2R1B,IMP3andGSTM2as candidate breast cancer susceptibility genes. Regional association plots for the remaining eight gene- based associations are provided in Supplementary Figure2 When we considered information from all eQTL associated with disease risk for each of the 11 genes (Supplementary Data 11 ), we found that decreased disease risk was consistently associated with decreased gene expression for three genes and increased expression for five genes (Table 3 and Supplementary Data 12 ). For the remaining three genes, inconsistent directional effects were observed across different eQTL. Table 3 Directional effect of genetically determined gene expression on disease risk for genes identified in the gene-based analysis of the adjusted breast cancer GWAS Full size table Lastly, we used EUGENE to determine if any of the 88 target genes of sentinel risk variants identified based on individual eQTL also had a significant gene-based association in the adjusted GWAS results. This would indicate that information from additional breast cancer risk variants (i.e. in low LD with the sentinel risk variants) supported the original target gene prediction, which could be used to prioritize genes for functional follow-up. We found that 11 of the 88 target genes had a nominally significant gene-based association in the adjusted GWAS results (EUGENE P < 0.05; Supplementary Data 13 ), with one remaining significant after correcting for multiple testing: CBX6 (EUGENE P = 0.0002). Estrogen receptor (ER)-negative breast cancer We applied the same analyses described above to results from the Milne et al. GWAS of ER-negative breast cancer, which included data on 21,468 cases and 100,594 controls, combined with 18,908 BRCA1 mutation carriers (9414 with breast cancer) [3] . Of the 54 sentinel risk variants identified through approximate joint association analysis (Supplementary Data 14 ), 19 were in LD ( r 2 > 0.8) with a sentinel eQTL (Supplementary Data 15 ), implicating 24 genes as likely targets of risk-associated variants for ER-negative breast cancer (Supplementary Data 16 ). Of these, 13 were also identified as likely targets of variants associated with overall breast cancer risk, while the remaining 11 genes were specific to ER-negative risk variants: ATM , CCNE1 , CUL5 , MCHR1 , MDM4 , NPAT , OCEL1 , PIK3C2B , RALB , RP5-855D21 . 3 , and WDR43 . Seventeen genes were not highlighted as candidate target genes in the Milne et al. GWAS [3] (Supplementary Data 16 and Supplementary Data 17 ), mostly (15 genes) because they are predicted targets of risk variants identified in previous GWAS, which were not considered by Milne et al. [3] . The two exceptions were RP5-855D21 . 3 and CUL5 , identified in our study based on eQTL from adipose tissue and whole-blood, respectively. Regional association plots for the 17 genes that represent previously unreported predictions are presented in Supplementary Fig. 3 , with three examples shown in Fig. 4 . Fig. 4 Examples of previously unreported target gene predictions at known ER- negative breast cancer risk loci. Variants are represented by points colored according to the LD with the sentinel risk variant (red: ≥0.8, orange: 0.6–0.8, green: 0.4–0.6, light blue: 0.2–0.4, and dark blue: <0.2). Sentinel risk variants (triangles) were identified based on joint association analysis [9] . Figure shows on the y -axis the evidence for ER-negative breast cancer association (−log 10 of the P -value in the original published GWAS results [3] , obtained in that study using an inverse-variance meta-analysis), and on the x -axis chromosomal position. Gene structures from GENCODE v19 gene annotations are shown and the predicted target genes shown in red. The sentinel risk variants are in LD with sentinel eQTL for MDM4 and PIK3C2B ( a ), ZNF703 ( b ), and ATM ( c ; Supplementary Data 17 ). 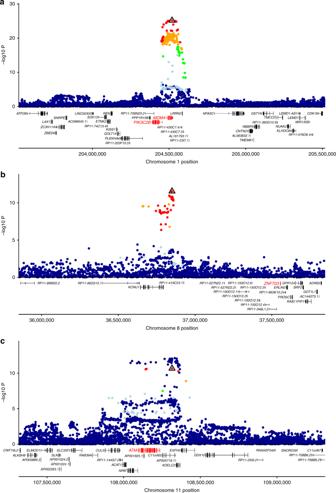Fig. 4 Examples of previously unreported target gene predictions at known ER- negative breast cancer risk loci. Variants are represented by points colored according to the LD with the sentinel risk variant (red: ≥0.8, orange: 0.6–0.8, green: 0.4–0.6, light blue: 0.2–0.4, and dark blue: <0.2). Sentinel risk variants (triangles) were identified based on joint association analysis9. Figure shows on they-axis the evidence for ER-negative breast cancer association (−log10of theP-value in the original published GWAS results3, obtained in that study using an inverse-variance meta-analysis), and on thex-axis chromosomal position. Gene structures from GENCODE v19 gene annotations are shown and the predicted target genes shown in red. The sentinel risk variants are in LD with sentinel eQTL forMDM4andPIK3C2B(a),ZNF703(b), andATM(c; Supplementary Data17). Regional association plots for the remaining 14 previously unreported target gene predictions are provided in Supplementary Figure3 Regional association plots for the remaining 14 previously unreported target gene predictions are provided in Supplementary Figure 3 Full size image The disease protective allele was associated with lower gene expression for seven genes and higher gene expression for 11 genes (summary in Table 4 and Supplementary Data 18 ; detailed information in Supplementary Data 15 ); for the remaining six genes, directional effect was either not available ( ATM , CASP8 , OCEL1 , PEX14 and WDR43 ) or inconsistent across tissues ( ADCY3 ). Table 4 Directional effect of genetically-determined gene expression on disease risk for predicted target genes of ER-negative breast cancer sentinel risk variants Full size table Of the 24 target gene predictions, 18 were supported by the presence of enhancer– promoter chromatin interactions or an association between enhancer epigenetic marks and gene expression (Supplementary Data 19 ). When we applied EUGENE to the ER-negative GWAS results obtained after conditioning on the 54 sentinel risk variants, we identified four genes in four loci with a significant gene-based association (EUGENE P < 2.5 × 10 −6 ; Table 5 , Supplementary Data 20 and Supplementary Fig. 4 ). Of these, we found that lower disease risk was consistently associated with lower expression for two genes ( VPS52 , GTF2IRD2B ) and higher expression for one gene ( INHBB ). For the fourth gene ( TNFSF10 ), directional effect was inconsistent across sentinel eQTL (detail and summary in Supplementary Tables 21 and 22 , respectively). Table 5 Risk loci for ER-negative breast cancer identified in the EUGENE gene-based analysis and not in previous GWAS Full size table Other genes that could be prioritized for functional follow-up include four (of the 24) target genes of sentinel risk variants that had a nominally significant gene-based association in the adjusted GWAS results (EUGENE P < 0.05; Supplementary Data 23 ): RALB , CCDC170 , NPAT , and CASP8 . Known role of the identified genes in cancer biology We used OncoScore, a text-mining tool that ranks genes according to their association with cancer based on available biomedical literature [21] , to assess the extent to which each of the breast cancer genes we identified were already known to have a role in cancer. Of the 112 genes we identified across the overall and ER-negative analyses that could be scored by OncoScore, 48 scored below the recommended OncoScore cut-off threshold (21.09) for novelty, including 25 with an OncoScore of 0, indicating no prior evidence for a role in cancer biology (Tables 2 and 5 ; Supplementary Tables 3 and 16 ). For the remaining 64 genes there is an extensive literature on their role in cancer, and breast cancer in particular. To predict candidate target genes at breast cancer risk loci, we identified sentinel eQTL in multiple tissues that were in high LD ( r 2 > 0.8) with sentinel risk variants from our recent GWAS [2] . Using this approach, we implicated 88 genes as likely targets of the overall breast cancer risk variants. Because eQTL are widespread, it is possible that some target gene predictions are false-positives due to coincidental overlap between sentinel eQTL and sentinel risk SNPs. At the LD threshold used, statistical methods developed recently to formally test for co-localization between eQTL and risk SNPs are of limited use, due to a high false-positive rate [22] . The 88 genes identified therefore represent target predictions that must be validated by functional studies. Of these 88, 26 genes had not been predicted as targets using a different approach that considered breast-specific functional annotations and eQTL data [2] , and so were considered previously unreported candidate target genes. Of the 26 previously unreported target predictions, all but one were identified from eQTL analyses in blood, spleen, or immune cells. They include several genes with a known role in immunity, including: HLF , the expression of which is associated with the extent of lymphocytic infiltration after neo-adjuvant chemotherapy [23] ; PTPN22 , a shared autoimmunity gene [24] , which encodes a protein tyrosine phosphatase that negatively regulates presentation of immune complex-derived antigens [25] ; and RHBDD3 , a negative regulator of TLR3-triggered natural killer cell activation [26] , and critical regulator of dendritic cell activation [27] . In addition, we identified IRF1 , which encodes a tumor suppressor and transcriptional regulator serving as an activator of genes involved in both innate and acquired immune response [28] , [29] , as a previously unreported breast cancer risk locus. These results suggest that at least some of the previously unreported predicted target genes play a role in cancer cell elimination or inflammation. However, another possibility is that eQTL detected in well-powered studies of blood are predictors of eQTL in other less accessible tissues, including breast and adipose tissue. Consistent with this possibility, about 50% of the eQTL found to be in LD with a sentinel risk variant for overall breast cancer (and similarly for ER-negative breast cancer) were associated with the expression of the respective target gene in the relatively small GTEx breast tissue dataset, although not at the conservative threshold that we used to define sentinel eQTL. Of note, one previously unreported target was identified through eQTL analyses in adipose tissue: ZNF703 . ZNF703 is a known oncogene in breast cancer [30] , and has been reported to be associated with breast size [31] which might suggest a role in adiposity. Using the same approach, we also identified 24 genes as likely targets of 19 ER- negative risk variants, of which 17 were not proposed as candidate target genes in the original GWAS [3] . Eleven of these 22 genes were unique to ER-negative breast cancer, including for example CUL5 , a core component of multiple SCF-like ECS (Elongin-Cullin 2/5-SOCS-box protein) E3 ubiquitin-protein ligase complexes which recognize proteins for degradation and subsequent Class I mediated antigen presentation [32] . We also identified previously unreported breast cancer risk loci using the recently described EUGENE gene-based association test [6] , [7] , which was developed to aggregate evidence for association with a disease or trait across multiple eQTL. Unlike other similar gene-based methods (e.g. S-PrediXcan), EUGENE includes in a single test information from eQTL identified in multiple tissues; this property is expected to increase power to detect gene associations when multiple cell types/tissues contribute to disease pathophysiology, for two main reasons. First, because tissue-specific eQTL are common, and so a multi-tissue analysis is able to capture the association between all known eQTL and disease risk in a single test. Second, because in single-tissue analyses, one needs to appropriately account for testing multiple tissues, thereby decreasing the significance threshold required for experiment-wide significance, which decreases power. When we applied EUGENE to the overall breast cancer GWAS [2] , we identified 11 associated genes located in six previously unreported risk loci. For most of these genes, there were multiple sentinel eQTL associated with overall breast cancer risk. In the analysis of ER-negative breast cancer [3] , EUGENE identified four associated genes ( INHBB, TNFSF10, VPS52 , and GTF2IRD2B ) located in four previously unreported risk loci. Some of the predicted target genes identified are well known to play a role in breast cancer carcinogenesis. For example, the genes identified for ER-negative breast cancer included MDM4 , encoding a negative regulator of TP53, which is necessary for normal breast development [33] ; CCNE1 , an important oncogene in breast cancer [34] , [35] ; CASP8 , encoding a regulator of apoptosis [36] ; ATM , a known breast cancer susceptibility gene [37] , [38] ; and the ER, ESR1 , which encodes a critical transcription factor in breast tissue [39] . On the other hand, the 11 significant gene-based associations for overall breast cancer included GSTM2 , which is part of the mu class of glutathione S-transferases that are involved in increased susceptibility to environmental toxins and carcinogens [40] . Other noteworthy gene-based associations included those with: IMP3 , which contributes to self-renewal and tumor initiation, properties associated with cancer stem cells [41] ; PPP2R1B , which encodes the beta isoform of subunit A of Protein Phosphatase 2A, itself a tumor suppressor involved in modulating estrogen and androgen signaling in breast cancer [42] ; and SEMA4A [43] , recently shown to regulate the migration of cancer cells as well as dendritic cells [44] . Two recent studies reported results from analyses that are similar in scope to those carried out in our study. First, Hoffman et al. [45] reported that genetically determined expression of six genes was associated with risk of breast cancer: three when considering expression in breast tissue ( RCCD1 , DHODH , and ANKLE1 ) and three in whole blood ( RCCD1 , ACAP1 , and LRRC25 ). Of note, RCCD1 and LRRC25 were identified as likely targets of known breast cancer risk variants in our analysis. We also found some support for an association between breast cancer risk and eQTL for ACAP1 (EUGENE P = 0.003) and ANKLE1 (EUGENE P = 0.01), but not for DHODH (best sentinel eQTL P = 0.119). Second, we recently applied a different gene-based approach called S-PrediXCan to results from the overall breast cancer GWAS [2] , using gene expression levels predicted from breast tissue [20] . This study reported significant associations with 46 genes ( P < 5.82 × 10 −6 ), including 13 located in 10 regions not yet implicated by GWAS. A major difference between our analyses is that the latter were based on the original GWAS summary statistics, without adjusting for the effects of the sentinel risk variants. This explains why most associated genes in their main analysis were located near known breast cancer risk variants. Of the 13 genes located in previously unreported risk loci, eight were tested in our analysis (which considered eQTL identified in multiple tissues, not just from breast as in ref. [20] ), of which four had a nominally significant ( P < 0.05) gene-based association: MAN2C1 ( P = 1.9 × 10 −6 ), SPATA18 ( P = 0.004), B3GNT1 ( P = 0.012), and CTD-2323K18 . 1 ( P = 0.021). These results show that at least four of the associations reported by Wu et al. [20] , which were based on information from breast eQTL only, are reproducible when a different gene-based approach is applied to the same GWAS results. Conversely, we identified a significant association with 13 genes not reported by Wu et al. [20] , all with a gene-based association driven by eQTL identified in non-breast tissues, mostly in immune cells and/or whole-blood. For 78 of the 114 genes that we implicate in breast cancer risk, either through target gene prediction or gene-based analyses, we were able to determine the directional effect of the breast cancer protective alleles on gene expression. In some cases, this was consistent with their known function. For example, ZNF703 is a well-known oncogene in breast cancer [30] and decreased expression was associated with decreased risk. Similarly, oncogenic activity has been reported for PIK2C2B [46] , for which we found that decreased expression is associated with decreased risk. Another gene for which decreased expression was associated with decreased risk was PTPN22 which is known to negatively regulate antigen presentation [47] and therefore might suppress immunoelimination. By contrast, CCNE1 [48] and APOBEC3A [49] have been reported to have oncogenic roles, but we found that increased expression was associated with decreased risk. We have previously found the same counterintuitive relationship between breast cancer risk alleles and CCND1 expression [50] . However, the expression patterns observed in breast tumors may not be relevant to the activity of these genes in the progenitor cells that give rise to breast tumors. The directional effect of genetically determined gene expression on breast cancer risk is important because drugs that mimic the effect of the protective allele on gene expression might be expected to attenuate (rather than exacerbate) disease risk. For example, decreased risk of ER-negative breast cancer was associated with decreased expression of KCNN4 , suggesting that an antagonist that targets this potassium channel and has a good safety profile [51] might reduce disease risk. Given these results, we suggest that KCNN4 should be prioritized for functional and pre-clinical follow up. In summary, we have used the largest available GWAS of breast cancer, along with expression data from multiple different tissues, to identify 26 and 17 previously unreported likely target genes of known overall and ER-negative breast cancer risk variants, respectively. We also describe significant gene-based associations at six and four previously unreported risk loci for overall and ER-negative breast cancer, respectively. Further investigation into the function of the genes identified in breast and immune cells, particularly those which have additional support from experimental or computational predictions of chromatin looping, should provide additional insight into the etiology of breast cancer. Predicting target genes of breast cancer risk variants Recently, Michailidou et al. [2] reported a breast cancer GWAS meta-analysis that combined results from 13 studies: the OncoArray study (61,282 cases and 45,494 controls); the iCOGS study (46,785 cases and 42,892 controls); and 11 other individual GWAS (with a combined 14,910 cases and 17,588 controls). That is, a total of 122,977 cases and 105,974 controls. The first aim of our study was to identify likely target genes of breast cancer risk variants identified in that GWAS. First, we identified variants associated with variation in gene expression (i.e. eQTL) in published transcriptome studies of five broad tissue types: adipose, breast, immune cells isolated from peripheral blood, spleen and whole- blood. We identified a total of 35 transcriptome studies reporting results from eQTL analyses in any one of those five tissue types (Supplementary Data 2 ). Some studies included multiple cell types and/or experimental conditions, resulting in a total of 86 separate eQTL datasets. For each eQTL dataset, we then (i) downloaded the original publication tables containing results for the eQTL reported; (ii) extracted the variant identifier, gene name, association P -value and, if available, the effect size (specifically, by “effect size” we mean the beta/ z -score) and corresponding allele; (iii) excluded eQTL located >1 Mb of the respective gene (i.e. trans eQTL), because often these are thought to be mediated by cis effects [52] ; (iv) excluded eQTL with an association P > 8.9 × 10 −10 , a conservative threshold that corrects for 55,764 transcriptsin Gencode v19, each tested for association with 1000 variants (as suggested by others [53] , [54] , [55] ); and (v) for each gene, used the --clump procedure in PLINK to reduce the list of eQTL identified (which often included many correlated variants) to a set of ‘sentinel eQTL’, defined as the variants with strongest association with gene expression and in low LD ( r 2 < 0.05, linkage disequilibrium (LD) window of 2 Mb) with each other. Second, we identified variants that were independently associated with breast cancer risk at a P < 5 × 10 −8 in the GWAS reported by Michailidou et al. [2] , which included 122,977 cases and 105,974 controls. We refer to these as “sentinel risk variants” for breast cancer. To identify independent associations, we first excluded from the original GWAS (which tested 12,396,529 variants) variants with: (i) a sample size < 150,000; (ii) a minor allele frequency < 1%; (iii) not present in, or not polymorphic (Europeans) in, or with alleles that did not match, data from the 1000 Genomes project (release 20130502_v5a); and (iv) not present in, or with alleles that did not match, data from the UK Biobank study [56] . After these exclusions, results were available for 8,248,946 variants. Next, we identified sentinel risk variants using the joint association analysis (--cojo- slct) option of GCTA [9] , using imputed data from 5000 Europeans from the UK Biobank study [56] to calculate LD between variants. These individuals were selected based on the sample IDs (lowest 5000) from our approved UK Biobank application 25331. Third, we identified genes for which a sentinel eQTL reported in any of the 86 eQTL datasets described above was in high LD ( r 2 > 0.8) with a breast cancer sentinel risk variant. That is, we only considered genes for which there was high LD between a sentinel eQTL and a sentinel risk variant, which reduces the chance of spurious co-localization. Directional effect of gene expression on breast cancer risk Having identified a list of genes with expression levels correlated with sentinel risk variants, we then studied the directional effect of the breast cancer protective allele on gene expression. For each sentinel eQTL in high LD ( r 2 > 0.8) with a sentinel risk variant, we: (i) identified the allele that was associated with reduced breast cancer risk, based on results reported by Michailidou et al. [2] ; and (ii) determined if that allele was associated with increased or decreased target gene expression in each of the eQTL datasets that reported that eQTL. For many studies, the directional effect of eQTL (i.e. effect allele and beta) was not publicly available, and so for those this analysis could not be performed. We also assessed whether the directional effect of gene expression on disease risk predicted by the approach described in the previous paragraph, which considered one eQTL at a time (a limitation) but many different eQTL datasets (a strength), would be recapitulated by applying S-PrediXcan [10] to the same breast cancer GWAS [2] using transcriptome information from 922 whole-blood samples studied by Battle et al. [11] . S-PrediXcan considers information from multiple eQTL identified for a given gene in a given tissue (e.g. whole-blood) when determining the association between genetically determined gene expression levels and disease risk. Therefore, we reasoned that this approach could be particularly useful for genes with multiple independent eQTL identified in the same tissue. The limitation of this approach is that it first requires the generation of gene expression prediction models based on individual-level variant and transcriptome data, which are not publicly available for most of the 35 transcriptome studies included in our analysis. We used gene expression models generated based on the whole-blood dataset of Battle et al. [11] because (i) most likely target genes were identified in our study based on eQTL information from whole-blood or immune cells isolated from whole-blood; and (ii) this was the largest transcriptome dataset we had access to. Target gene predictions supported by functional data Sentinels and variants in high LD ( r 2 > 0.8 in Europeans of the 1000 Genomes Project, with MAF > 0.01) were queried against the following sources of publicly available data generated from blood-derived samples and cell lines. Computational methods linking regulatory elements with target genes including PreSTIGE [17] , FANTOM5 [16] , IM-PET [18] , enhancers and super enhancers from Hnisz et al. [19] . Experimental chromatin looping data defined by ChIA-PET [13] and capture Hi-C [4] , [14] and in situ Hi-C [15] were mined to identify physical interactions between query SNPs and target gene promoters. Variants were assigned to potential target genes based on intersection with associated enhancer annotations using BedTools intersect [57] . Identification of previously unreported risk loci for breast cancer The second aim of this study was to use a gene-based approach to identify loci containing breast cancer risk variants that were missed by the single-variant analyses reported by Michailidou et al. [2] . At least three gene-based approaches have been described recently to combine in a single test the evidence for association with a disease across multiple eQTL [6] , [8] , [10] . Of these, we opted to use EUGENE [6] , [7] because it is applicable to GWAS summary statistics and combines in the same association test information from eQTL identified in different tissues and/or transcriptome studies. The latter feature is important for two main reasons. First, because multiple tissue types are likely to play a role in the pathophysiology of breast cancer, and tissue-specific eQTL are common [58] . Second, because different transcriptome studies of the same tissue (e.g. blood) identify partially (not completely) overlapping lists of eQTL. This might arise, for example, because of differences in sample size, gene expression quantification methods (e.g. microarrays vs. RNA-seq, data normalization) or demographics of the ascertained individuals (e.g. age, disease status). Therefore, identifying eQTL based on information from multiple tissues and/or studies is expected to produce a more comprehensive list of regulatory variants that could be relevant to breast cancer pathophysiology. An additional advantage of EUGENE is that it considers in the same test different types of eQTL (e.g. with exon-specific or stimulus-specific effects), thereby increasing the likelihood that causal regulatory variants related to breast cancer are captured in the analysis [59] . EUGENE requires an input file that lists all eQTL that will be included in the gene- based test for each gene. To generate such list for this study, we did as follows for each gene in the genome. First, we took the union of all eQTL reported in the 86 eQTL datasets described above. Second, we used the --clump procedure in PLINK to reduce the list of reported eQTL to a set of ‘sentinel eQTL’, defined as the variants with strongest association with gene expression and in low LD ( r 2 < 0.1, LD window of 1  Mb) with each other. Note that clumping was not performed separately for each tissue or study, but rather applied to the union of eQTL identified across all tissues/studies. If an eQTL was identified in multiple tissues/studies, the clumping procedure was performed using the smallest P -value reported for that eQTL across all tissues/studies. A file (BREASTCANCER.20170517.eqtl.proxies.list) containing the sentinel eQTL identified per gene is available at [ https://genepi.qimr.edu.au/staff/manuelF/eugene/main.html ]. For each gene, EUGENE extracts single-variant association results for each sentinel eQTL identified (or, if not available, for a proxy with r 2 > 0.8) from the GWAS summary statistics, sums the association chi-square values across those eQTL, and estimates the significance (i.e. P -value) of the resulting sum test statistic using Satterthwaite's approximation, which accounts for the LD between eQTL [7] . This approximation was originally implemented by Bakshi et al. [60] in the GCTA-fastBAT module and is now also available in EUGENE. LD between eQTL was estimated based on data from 294 Europeans from the 1000 Genomes Project (release 20130502_v5a). Because our aim was to identify previously unreported breast cancer risk loci, we did not apply EUGENE to the original results reported by Michailidou et al. [2] . Had we done so, significant gene-based associations would have been disproportionally located in known risk loci; associations driven by previously unreported risk variants would therefore be more difficult to highlight. Instead, we first adjusted the results [2] for the effects of the sentinel risk variants identified (see section above), using the --cojo-cond option of GCTA [9] . In doing so, we obtained adjusted GWAS results with no single variant with an association P < 5 × 10 −8 . We then applied EUGENE to the adjusted GWAS results, including a correction of the single-variant association statistic (i.e. chi-square) for an LD-score regression intercept [61] of 1.1072. This correction was important to account for the inflation of single-variant test statistics observed in Michailidou et al. [2] that were likely due to unaccounted biases. To maintain the overall false-positive rate at 0.05, the significance threshold required to achieve experiment-wide significance in the gene-based analysis was set at P < 0.05/ N genes tested. OncoScore We used OncoScore, a text-mining tool that ranks genes according to their association with cancer based on available biomedical literature [21] , to determine which of the breast cancer genes we identified were already known to have a role in cancer. ER-negative breast cancer Lastly, we used the approaches described above to identify target genes and previously unreported risk loci for ER-negative breast cancer. In this case, single-variant summary association statistics were obtained from the Milne et al. [3] GWAS, which included 21,468 ER-negative cases and 100,594 controls from the Breast Cancer Association Consortium, combined with 18,908 BRCA1 mutation carriers (9414 with breast cancer) from the Consortium of Investigators of Modifiers of BRCA1/2 , all tested for 17,304,475 variants (9,827,195 after the exclusions described above). The LD-score regression intercept used to correct the single-variant association statistics of this GWAS was 1.0637. Study approval Informed consent was obtained from all subjects participating in the Breast Cancer Association Consortium under the approval of local Institutional Review Boards. Ethics approval was obtained from the Human Research Ethics Committee of QIMR-Berghofer.